Topological crystalline insulators in the SnTe material class Topological crystalline insulators are new states of matter in which the topological nature of electronic structures arises from crystal symmetries. Here we predict the first material realization of topological crystalline insulator in the semiconductor SnTe by identifying its non-zero topological index. We predict that as a manifestation of this non-trivial topology, SnTe has metallic surface states with an even number of Dirac cones on high-symmetry crystal surfaces such as {001}, {110} and {111}. These surface states form a new type of high-mobility chiral electron gas, which is robust against disorder and topologically protected by reflection symmetry of the crystal with respect to {110} mirror plane. Breaking this mirror symmetry via elastic strain engineering or applying an in-plane magnetic field can open up a continuously tunable band gap on the surface, which may lead to wide-ranging applications in thermoelectrics, infra-red detection and tunable electronics. Closely related semiconductors PbTe and PbSe also become topological crystalline insulators after band inversion by pressure, strain and alloying. The discovery of topological insulators [1] , [2] , [3] has attracted much interest in topological states of matter beyond the existing Z 2 material class. In searching for new phases, crystal symmetries have a multifaceted role by either constraining the band topology [4] , [5] or engendering new ones [7] , [8] . Topological crystalline insulators [8] are such new states of matter in which the topological nature of electronic structures arises from crystal symmetries. Thanks to the complexity and richness of crystal structures, the study of topological crystalline insulators has just begun and a large number of topological crystalline insulators awaits discovery—both theoretically and experimentally. In this work, we theoretically demonstrate that SnTe is a topological crystalline insulator with mirror symmetry. As a consequence, it is predicted to have robust surface states with an even number of Dirac cones on crystal surfaces such as {001}, {110} or {111}, which are symmetric about {110} mirror planes. The notation {hkl} refers to the (hkl) plane and all those that are equivalent to them by virtue of the crystal symmetry (a similar convention is used with directions: n 1 n 2 n 3 refers to, collectively, the [ n 1 n 2 n 3 ] direction and its equivalent ones). The existence of these surface states is dictated by a non-zero integer topological invariant—the mirror Chern number [9] . Crystal structure and mirror symmetry SnTe has a simple rocksalt structure ( Fig. 1a ); its fundamental band gaps are located at four equivalent L points in the face-centered-cubic Brillouin zone. It has long been established that the ordering of the conduction and valence bands at L points in SnTe is inverted relative to PbTe, so that the band gap of the alloy Pb 1− x Sn x Te closes and re-opens as x increases [10] . As this band inversion occurs at an even number of points, neither SnTe nor PbTe in the rocksalt structure is a topological insulator with Z 2 topological order. 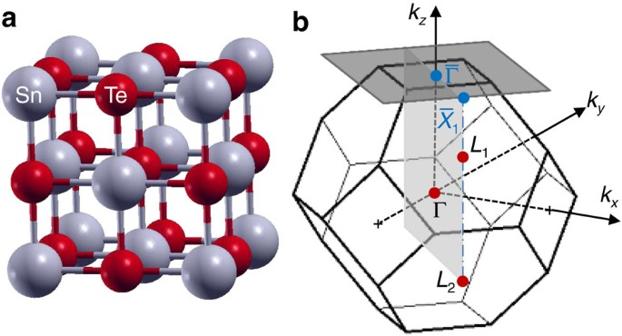Figure 1: SnTe lattice and Brillouin zone. (a) the crystal structure of SnTe; (b) the face-centered-cubic (FCC) Brillouin zone showing the plane ΓL1L2, which is invariant under reflection about the (110) axis and projects onto theline in the [001] surface. Figure 1: SnTe lattice and Brillouin zone. ( a ) the crystal structure of SnTe; ( b ) the face-centered-cubic (FCC) Brillouin zone showing the plane Γ L 1 L 2 , which is invariant under reflection about the (110) axis and projects onto the line in the [001] surface. Full size image However, the above band inversion has significant consequences when the mirror symmetry of the face-centered-cubic lattice is taken into consideration. Consider the plane Γ L 1 L 2 in momentum space, defined by the three points Γ, L 1 and L 2 ( Fig. 1b ). Crystal momenta on this plane are invariant under reflection about the {110} mirror planes in real space. This allows us to label the Bloch wavefunctions on this plane by their eigenvalues ± i under the mirror operation M (which satisfies M 2 =−1 for spin 1/2 electrons). Each class of M = ± i mirror eigenstates has an associated Chern number n ± i , and the mirror Chern number n M [9] is defined by n M =( n + i − n − i )/2. Provided that mirror symmetry is present, n M is an integer topological invariant. A non-zero mirror Chern number defines a topological crystalline insulator with mirror symmetry. Mirror Chern numbers of SnTe and PbTe We first demonstrate that SnTe and PbTe have mirror Chern numbers that differ by two, and hence, one of them is a topological crystalline insulator. This is established by considering the band inversion at four L points between SnTe and PbTe. The k·p theory of the band structure near a given L point is given by Mitchell and Wallis [11] : Here k 1 , k 2 , k 3 form an orthogonal system with k 3 along Γ L and k 1 along the [110] direction perpendicular to the mirror plane; σ z = ±1 corresponds to the p -orbital on the cation (Sn or Pb) and anion (Te), respectively; s 3 = ±1 labels the total angular momentum j =±1/2 along Γ L . A positive m means that the conduction and valence bands at L are respectively derived from the cation and anion, and vice versa for negative m . The form of H in equation (1) is uniquely determined by the D 3 d point group symmetries, which leave an L point invariant [12] . In particular, reflection about the (110) mirror plane is represented by M = − is 1 . On the mirror-invariant plane Γ L 1 L 2 ( k 1 =0), H reduces to . Due to mirror symmetry, H 0 decomposes into the s 1 =1 ( M =− i ) and s 1 =−1 ( M = i ) subspaces: each of which describes a two-dimensional massive Dirac fermion. In going from PbTe to SnTe (increasing x in Pb 1− x Sn x Te), the cation/anion character of the conduction/valence bands becomes switched at L , which in the k · p theory corresponds to m→ − m . The sign reversal of m at one L point changes the Chern number of the s 1 = ±1 subspace by ±1, and hence the mirror Chern number changes by one. Furthermore, L 1 and L 2 are related by a two-fold rotation around the axis. Under this rotation, both the spin polarization s 1 and the orientation of the Γ L 1 L 2 plane are flipped. As a result, the Berry curvatures at L 1 and L 2 are related by so that that is, both L 1 and L 2 contribute equally to the change in mirror Chern number. The net result is that the band inversion changes the mirror Chern number for the Γ L 1 L 2 plane by two. From this, we deduce that SnTe and PbTe are topologically distinct phases, as long as the reflection symmetry with respect to any of the six equivalent {110} mirror planes is present. SnTe is topologically non-trivial To determine which of the two is topologically non-trivial, we analyse their band structures obtained from first-principles density functional theory calculations [13] , [14] , [15] , [16] , [17] , [18] , using the generalized gradient approximation [19] . The results we obtain are consistent with several previous studies [20] , [21] , [22] , [23] . In particular, it is generally agreed that the band ordering at L points is correct at the total-energy optimized volume. On the basis of two first-principles findings, we now demonstrate that, of the two materials, SnTe is the topologically non-trivial one. First, the conduction and valence bands of PbTe throughout the Brillouin zone are primarily derived from the p -orbitals of Pb and Te atoms, respectively ( Fig. 2b ). This suggests that PbTe is smoothly connected to the atomic limit, in which Pb orbitals are empty and Te orbitals filled due to their on-site energy difference. In contrast, the orbitals in the band structure of SnTe are switched near L points: the conduction band edge is derived from Te and the valence band edge from Sn ( Fig. 2a ). Therefore, SnTe has an intrinsically inverted band structure ( m <0). Our conclusion is further supported by the dependence of the band gap on the lattice constant obtained in first-principles calculations ( Fig. 2c ) and measured via pressure co-efficients [24] . As the lattice constant increases, the band gap of PbTe increases monotonically, whereas that of SnTe decreases to zero and then re-opens. This gap closing signals a topological phase transition, in which SnTe at ambient pressure is a topological crystalline insulator with the aforementioned mirror Chern number n M = −2. The sign of n M has been discussed in detail in ref. 9 . 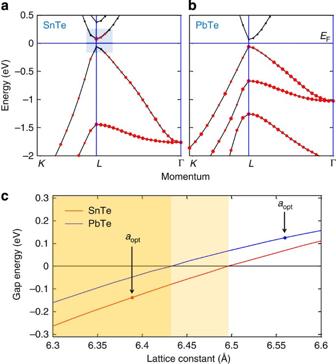Figure 2: Electronic structures and band-gap evolution of SnTe and PbTe. The electronic band structures of SnTe and PbTe are shown in (a) and (b), respectively. The size of the red dots represents the fraction of electronic charge residing on Te atoms. The exchange of the band character atLpoint as highlighted in the grey area indicates the intrinsic band inversion of SnTe. The band-gap energy as a function of the lattice constants is shown in (c). The negative gap area indicates the topological crystalline insulator phase. Figure 2: Electronic structures and band-gap evolution of SnTe and PbTe. The electronic band structures of SnTe and PbTe are shown in ( a ) and ( b ), respectively. The size of the red dots represents the fraction of electronic charge residing on Te atoms. The exchange of the band character at L point as highlighted in the grey area indicates the intrinsic band inversion of SnTe. The band-gap energy as a function of the lattice constants is shown in ( c ). The negative gap area indicates the topological crystalline insulator phase. Full size image Surface states of SnTe The non-zero mirror Chern number in SnTe dictates the existence of surface states on any crystal surface symmetric about the {110} mirror planes. Three common surface terminations satisfying this condition are: {001}, which is symmetric about two equivalent {110} mirror planes; {111}, which is symmetric about three equivalent mirror planes; and {110}, which is symmetric about the mirror plane. According to the bulk-boundary correspondence, we now infer the topology of these surface bands. For the {001} surface, the plane Γ L 1 L 2 in the bulk Brillouin zone projects onto the symmetry line in the surface Brillouin zone, with both L 1 and L 2 projecting onto . The mirror Chern number n M = −2 dictates that there must exist two pairs of counter-propagating, spin-polarized surface states with opposite mirror eigenvalues along the line . By rotational symmetry, such surface states also appear along the line . But they are absent along any other mirror-invariant line. The crossing of two mirror branches creates an anisotropic two-dimensional Dirac point with different velocities along the parallel and perpendicular direction. Therefore, the {001} surface states have four Dirac points located on the four equivalent lines. Similar considerations apply to the other two surfaces. For the {111} surface, the plane Γ L 1 L 2 projects onto the line ; so there are two Dirac points along each of the three equivalent lines . For the {110} surface, the plane Γ L 1 L 2 projects onto the line , on which there are two Dirac points. In all cases, surface states of SnTe have an even number of Dirac points, which can be easily distinguished from Z 2 topological insulators having an odd number. Our theoretical prediction of these surface states is the main result of this work. Using first-principles calculations, we now explicitly demonstrate the above surface states in a slab geometry along the [001] axis. Results for other surfaces will be published elsewhere. As predicted by the above topological band theory, two surface bands with opposite mirror eigenvalues are found to cross each other and form a Dirac point on the line ( Fig. 3a ). The Dirac velocity is found to be 1.7×10 5 m/s in the direction. Interestingly, these surface states exhibit a Lifshitz transition—a change of Fermi surface topology as a function of Fermi energy. 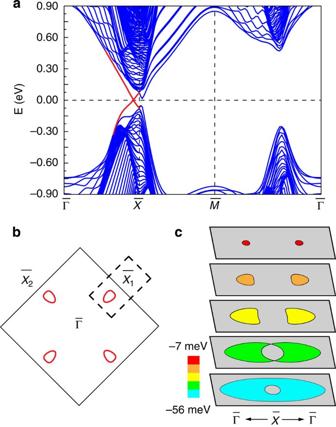Figure 3: The [001] surface states of SnTe. (a) band dispersion and (b) Fermi surface. Note that in betweenandtwo surface bands with opposite mirror eigenvalues cross the Fermi energy, in agreement withnM= −2. (c) a set of Fermi surfaces at different energies, exhibiting a Lifshitz transition. Figure 3b shows a set of Fermi surfaces at different energies. As the Fermi energy decreases from the Dirac point towards the valence band, the Fermi surface initially consists of two disconnected hole pockets outside ; the two pockets then touch each other and reconnect to form a large hole and a small electron pocket, both centred at . Figure 3: The [001] surface states of SnTe. ( a ) band dispersion and ( b ) Fermi surface. Note that in between and two surface bands with opposite mirror eigenvalues cross the Fermi energy, in agreement with n M = −2. ( c ) a set of Fermi surfaces at different energies, exhibiting a Lifshitz transition. Full size image To understand both the connection between the bulk and surface bands, and the effect of potential perturbations at a microscopic level, we introduce a simplified tight-binding model for SnTe, detailed in Methods. Using the tight-binding model, we now study the electronic properties of the {001} surface states under various perturbations. Similar analysis applies to other surfaces. The doubly degenerate surface states ψ α ( K j ) at the four Dirac points K j have opposite mirror eigenvalues i α, and hence opposite expectation values of spin polarization perpendicular to the K j direction. For convenience, we choose a natural basis in which the relative phases between the wavefunctions at different Dirac points are fixed by the four-fold rotation relating them In this basis, the k · p Hamiltonians at four Dirac points take an identical form: Here k 1 and k 2 form a local right-handed coordinate system centred at each K j , with k 2 parallel to K j . It is important to note that the four branches of surface Dirac fermions have the same chirality, defined by the relative sign of and v || in equation (6). As such, the surface states of the topological crystalline insulator SnTe form a “chiral” Dirac metal protected by crystal symmetries, thereby defining a new symmetry/topology universality class. In particular, provided that mirror symmetry is present ( k 1 → − k 1 , s 2 → − s 2 ), the Dirac points here line, but cannot annihilate with each other. We now consider ways to engineer a band gap on the surface. Perturbations which break mirror symmetries can generate Dirac mass term m j s 3 and thus open up energy gaps E j =2| m j | at the Dirac points. The nature of the gapped phase depends on the relative signs of m j , which is determined by the symmetry of the perturbation. For example, a perpendicular magnetic field B couples to electron's spin and yields Dirac masses of the same sign due to rotational invariance: m 1 = m 2 = m 3 = m 4 B . This drives the surface states into an integer quantum Hall state. The perturbations which break the four fold rotation symmetry of the {001} surface are particularly interesting. One example is a structure distortion with atoms being displaced by a vector u , which can be introduced by strain and possibly external electric field. Also, SnTe is known to spontaneously distort along the [111] direction into a rhombohedral structure at low temperature. This perturbation is time-reversal invariant but breaks rotational symmetry, leading to a ferroelectric phase. Although this distortion has negligible effect on the band structure in the bulk, it can dramatically affect the Dirac surface states. The effect of the distortion can be captured by adding a modulated hopping term to the tight binding model (see Methods). By symmetry analysis (equation (5)), one can show that the distortion gives the following anisotropic Dirac mass terms: where is the surface normal. As a result, the metallic surface acquires a band gap, which is linearly proportional to the magnitude of structural distortion and depends on its direction. For the rhombohedral distortion u [111], the two Dirac points along the direction are gapped, but the other two along the [110] direction remain gapless due to the unbroken (110) mirror plane. The ability to continuously tune the surface band gap via applying strain suggests potential electronic and optoelectronic device applications based on topological crystalline insulators such as SnTe. Likewise, an in-plane magnetic field in the u direction generates Dirac mass terms given by m j u · K j . In particular, when the magnetic field is perpendicular to one of the mirror planes, the system is still symmetric about this mirror plane and hence continues to exhibit gapless surface states despite the broken time reversal symmetry. Therefore, topological crystalline insulators defined by mirror Chern number also exist in magnetic systems such as Mn- and Cr-doped SnTe [25] ], contrary to existing Z 2 topological insulators. As equation (7) shows, when the displacement vector u points along the mirror invariant line , the surface states remain gapless at two Dirac points. Therefore, there are four distinct types of fully gapped surface ferroelectric phases depending on the direction of u ( Fig. 4 ). These ferroelectric phases correspond to breaking crystal symmetry in “different directions” and their electronic structures cannot be adiabatically connected. Now consider two such gapped ferroelectric regions (A and B), which are spatially adjacent to each other. The domain wall between them turns out to be particularly interesting if u A lies in the I–III quadrants and u B the II-IV quadrants. Owing to their different displacement vectors, a pair of Dirac masses at opposite momenta change sign in going from A to B. As a result, there exists a time-reversed pair of counter-propagating one-dimensional gapless states bound to the domain wall. Similar to the edge states of quantum spin Hall insulators, the domain wall states here are protected from elastic backscattering [26] , and form perfectly conducting channels. 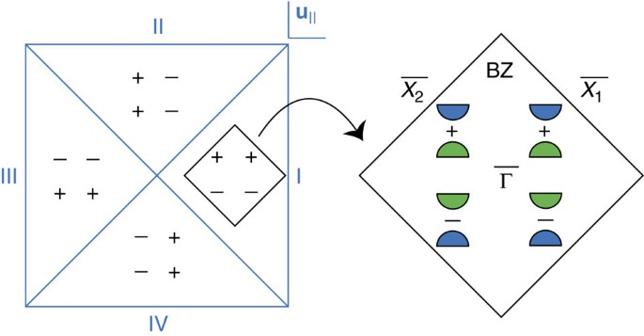Figure 4: The four surface ferroelectric phases, each with the signs of the Dirac masses. Under a ferroelectric distortion with a displacementu, the four surface Dirac points (detailed on the right) are gapped with mass signs depending on the direction ofu||. This leads to the four gapped phases (I–IV). Figure 4: The four surface ferroelectric phases, each with the signs of the Dirac masses. Under a ferroelectric distortion with a displacement u , the four surface Dirac points (detailed on the right) are gapped with mass signs depending on the direction of u || . This leads to the four gapped phases (I–IV). Full size image The existence of such domain wall states explains the robustness of these surface states against time-reversal-invariant disorder. By definition, disorder breaks mirror symmetry in a random way locally, not macroscopically. For the sake of argument, let us assume that the disorder potential is slowly varying. The surface is then an equal-weight mixture of the aforementioned type I–III and type II–IV ferroelectric domains, with domain walls percolating throughout the surface. As the domain wall is a perfectly conducting channel, the entire surface must be conducting. A similar situation occurs in disordered weak topological insulators [27] , [28] , [29] . The above analysis of disorder also accounts for surface roughness. Surfaces without any symmetry are generically gapped. Similar to structural distortions, different crystal faces correspond to breaking crystal symmetry in different directions. By the same reasoning, the aforementioned one-dimensional domain wall states exist on edges connecting them. As a result, a surface is guaranteed to be metallic, if it preserves mirror symmetry on average in the sense of exhibiting sharp Bragg diffraction peaks as the clean surface. A comprehensive theory of disordered topological crystalline insulators is in progress. On the experimental side, the surface states of SnTe we predicted can be readily detected in angle-resolved photoemission spectroscopy and tunnelling spectroscopy experiments. The underlying mirror Chern number can be deduced from the spin polarization of surface states [30] . Moreover, SnTe-based thin films and superlattices have remarkably high mobility, exceeding 2500 cm 2 /Vs at room temperature [31] , [32] , which provide a promising platform for device applications. Finally, we relate our work to a wider class of materials, including PbTe and PbSe. Although both are topologically trivial at ambient pressure, our first-principles calculation ( Fig. 2c ) shows that decreasing the lattice constant by 2% inverts the band gap and drives PbTe into a topological crystalline insulator. This band inversion is realized under moderate pressure (around 3 GPa in PbTe and 2 GPa in PbSe [24] , [22] ). Alternatively, one can achieve the topological regime by growing these materials on substrates with smaller lattice constants. As a precedent, high-quality PbTe quantum wells have been fabricated and exhibit ballistic transport [33] , [34] . It is also known that the alloys Pb 1− x Sn x Te and Pb 1− x Sn x Se undergo band inversion as Sn composition increases [35] , [36] , so that they become topological crystalline insulators on the inverted side. We briefly comment on how our work relates to early pioneering field-theoretic studies, which predicted the existence of two dimensional massless Dirac fermions at the interface of PbTe and SnTe [37] , [38] , or domain wall of PbTe [39] . Our work has made it clear that only interfaces symmetric about the {110} mirror plane have protected gapless states, which are solely derived from the topological crystalline insulator SnTe and exist even when PbTe is removed. In light of ther topological nature, which we identified, SnTe material class in IV–VI semiconductors is likely to lead a new generation of topological materials. Tight binding model The tight-binding model for SnTe is constructed from the Wannier functions of the conduction and valence bands, which are primarily three p -orbitals of Sn and Te atoms. The Hamiltonian H tb is given by Here r labels the site, j =1,2 labels the Sn or Te atom, α =↑,↓ labels electron's spin. The components of vectors c † and c correspond to the three p -orbitals. In the Hamiltonian (equation (8)), m is the on-site potential difference between Sn and Te; t 12 = t 21 is the nearest-neighbour hopping amplitude between Sn and Te; t 11 and t 22 are the next nearest-neighbour hopping amplitudes within a sublattice; is the unit vector connecting site r to r ′. The second line thus represents σ-bond hopping (head-to-tail) of the p -orbitals. The λ 1,2 term is L · s atomic spin-orbit coupling, where is the orbital angular momentum in p -orbital basis. The bulk and surface bands of the above tight-binding Hamiltonian nicely reproduce the essential features of the first-principles calculation, and additional terms such as π-bond hopping of the p -orbitals can be added to improve the fit. The effect of a structural distortion in which atoms are displaced by u can be captured by adding the modulated hopping to the tight binding model. How to cite this article: Hsieh, T.H. et al . Topological crystalline insulators in the SnTe material class. Nat. Commun. 3:982 doi: 10.1038/ncomms1969 (2012).